Charge state manipulation of qubits in diamond The nitrogen-vacancy (NV) centre in diamond is a promising candidate for a solid-state qubit. However, its charge state is known to be unstable, discharging from the qubit state NV − into the neutral state NV 0 under various circumstances. Here we demonstrate that the charge state can be controlled by an electrolytic gate electrode. This way, single centres can be switched from an unknown non-fluorescent state into the neutral charge state NV 0 , and the population of an ensemble of centres can be shifted from NV 0 to NV − . Numerical simulations confirm the manipulation of the charge state to be induced by the gate-controlled shift of the Fermi level at the diamond surface. This result opens the way to a dynamic control of transitions between charge states and to explore hitherto inaccessible states, such as NV + . The nitrogen-vacancy (NV) centre in diamond has drawn considerable interest over the past years in such diverse fields like quantum information processing [1] , [2] , [3] , [4] , single-spin magnetometry [5] , [6] and plasmonics [7] , [8] . Most of these applications exploit the fact that the spin state of the negatively charged NV centre (NV − ) can be initialized and read out optically. However, this state has been observed to become unstable, turning into the neutral charge state NV 0 under various kinds of laser illumination [9] , [10] , [11] , close to the surface [12] , [13] , [14] , [15] or at high implantation densities [16] , [17] . For the engineering [18] , [19] , [20] of large-scale quantum processors [3] , [21] , it is therefore an outstanding goal to reliably control the charge state of an NV centre. This would not only enable stabilization of the NV − state but also allow to explore applications, which have been proposed for the neutral state [22] NV 0 . In addition, inaccessible states [23] such as NV + could be explored, and a dynamic control of transitions between charge states might be established. The charge state of defects in bulk semiconductors depends on the position of the Fermi level with respect to the defect's charge transition level, which is defined as the energy at which the defect takes up or loses an electron. For instance, the NV 0/− level marks the transition from the neutral to the negatively charged state. Thus, when the Fermi level is shifted above a charge transition level, an electron is taken up by the defect and vice versa. For NV centres in diamond, the NV 0/− charge transition level corresponds to the ground state of NV − , which is predicted to lie in the band gap 2.8 eV above the valence band maximum (VBM) [23] . The position of the NV +/0 level is expected to be below the NV 0/− level. A static chemical control of the charge state of NV colour centres in diamond has recently been shown [13] , [14] , [15] . For instance, control of the Fermi energy was achieved by exploiting surface transfer doping in hydrogen (H)-terminated diamond [24] . In this case, atmospheric adsorbates on the surface provide acceptor states for electrons from the diamond, which shift the Fermi level below the VBM. This renders the H-terminated surface conductive due to a two-dimensional hole gas, which is formed in the potential well at the surface. Moreover, the Fermi level is shifted below the charge transition levels of shallowly implanted NV centres, which then ionize from NV − into NV 0 and subsequently into a non-fluorescent state. We have previously shown that shallow implanted NV centres discharge below an oxygen (O)/hydrogen (H) patterned surface [14] . In this work, we demonstrate a method to dynamically manipulate the charge state of single NV centres with an electrolytic gate electrode. Similar to a diamond solution-gated field effect transistor [25] , an N + implanted and subsequently H-terminated diamond is immersed into an electrolyte and a gate voltage U G is applied between a reference electrode in the electrolyte (potential μ RE ) and the diamond surface ( Fig. 1a ). This voltage allows to electrically shift the Fermi level at the diamond surface ( Fig. 1b ), which, at the same time, also changes its surface band bending. Upon varying the gate voltage, single centres can be switched from an unknown non-fluorescent state into the neutral charge state NV 0 , and the population of an ensemble of centres can be shifted from NV 0 to NV − . 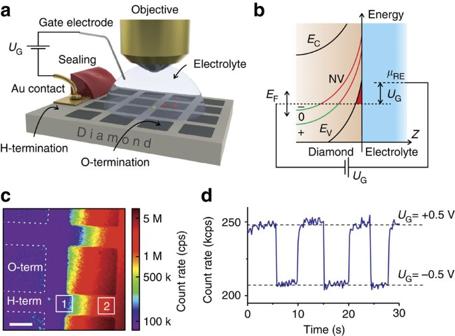Figure 1: Electrical manipulation of the charge state of NV centres in diamond. (a) Sketch of the experimental configuration showing the shallow-implanted NV centres in the O/H-patterned diamond surface. (b) Energy band schematic of the diamond/electrolyte interface. By applying a gate voltage between the gate electrode and H-terminated diamond, it is possible to control the Fermi energy level, moving it through the charge transition levels NV+/0and NV0/−. (c) Fluorescence image of an O/H-patterned diamond with shallow-implanted NV centres under floating gate conditions. Regions 1 and 2 indicate areas with low and high dose of NVs, respectively. (d) Time trace of the fluorescence intensity upon changes betweenUG=±0.5 V (650 nm longpass filter) recorded on region (2). Figure 1: Electrical manipulation of the charge state of NV centres in diamond. ( a ) Sketch of the experimental configuration showing the shallow-implanted NV centres in the O/H-patterned diamond surface. ( b ) Energy band schematic of the diamond/electrolyte interface. By applying a gate voltage between the gate electrode and H-terminated diamond, it is possible to control the Fermi energy level, moving it through the charge transition levels NV +/0 and NV 0/− . ( c ) Fluorescence image of an O/H-patterned diamond with shallow-implanted NV centres under floating gate conditions. Regions 1 and 2 indicate areas with low and high dose of NVs, respectively. ( d ) Time trace of the fluorescence intensity upon changes between U G =±0.5 V (650 nm longpass filter) recorded on region (2). Full size image Electrical control of the charge state in NV ensembles Experiments were conducted on electronic grade, synthetic, single-crystalline diamonds, with NV centres implanted at an average depth of 7 and 14 nm (5 and 10 keV implantation energy) [26] , where single optically resolved NV centres or densely implanted regions (regions 1 and 2 in Fig. 1c ) could be examined. Samples were patterned with O- and H-terminated regions (see Fig. 1c ). The conductive H-terminated surface was electrically contacted and the metal contacts isolated with silicone rubber. The sample was immersed in electrolyte, which was contacted by a platinum electrode. We investigated the effect of the gate voltage on the fluorescence in densely implanted H-terminated regions (nitrogen implantation dose around 10 13 cm −2 ) of the diamond surface (region 2 in Fig. 1c ). Figure 1d shows the fluorescence count rate in this region, recorded with a NV − —selective 650 nm longpass filter while the gate voltage is switched between +0.5 and −0.5 V. The NV fluorescence intensity decreases by about 20% during this change and is fully recovered when switching back to +0.5 V (see Fig. 1d ), suggesting that NV − centres are repeatedly discharged into NV 0 or potentially NV + . This is confirmed by optical spectra taken at both gate voltages ( Fig. 2a ). These spectra exhibit the characteristic emission of NV 0 (with a zero-phonon-line at 575 nm) and NV − (zero-phonon-line at 637 nm), and therefore allow to infer the populations of the NV 0 and NV − charge states. 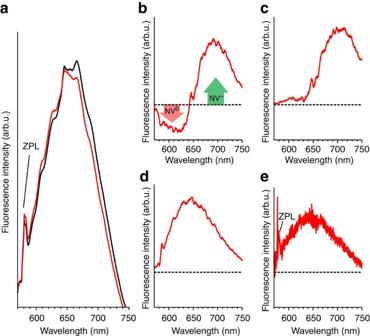Figure 2: Gate-dependent spectral properties of NV centres. (a) Spectra of the H-terminated area of a 10 keV implantation in a region with high implantation density (black:UG=+0.5 V, red:UG=−0.5 V). ZPL, zero-phonon-line. (b–d) Difference of the spectra atUG=+0.5 V andUG=−0.5 V ((b) at∼1013cm−2, (c) at∼1012cm−2and (d) at∼1011cm−2). The dashed line indicates zero level. (e) Difference spectrum of a single NV centre (implantation density∼1011cm−2) when switching fromUG=+0.4 V toUG=−0.4 V. The dashed line indicates zero level. Figure 2: Gate-dependent spectral properties of NV centres. ( a ) Spectra of the H-terminated area of a 10 keV implantation in a region with high implantation density (black: U G =+0.5 V, red: U G =−0.5 V). ZPL, zero-phonon-line. ( b – d ) Difference of the spectra at U G =+0.5 V and U G =−0.5 V (( b ) at ∼ 10 13 cm −2 , ( c ) at ∼ 10 12 cm −2 and ( d ) at ∼ 10 11 cm −2 ). The dashed line indicates zero level. ( e ) Difference spectrum of a single NV centre (implantation density ∼ 10 11 cm −2 ) when switching from U G =+0.4 V to U G =−0.4 V. The dashed line indicates zero level. Full size image The resulting change in the spectrum upon varying voltage is more clearly visible in Fig. 2b , which shows the difference between the spectra of Fig. 2a . Starting from a mixed population of negatively, neutrally and, potentially, positively charged NV centres, the amount of NV − increases at the expense of NV 0 when the gate voltage changes from −0.5 to +0.5 V. We tentatively interpret the relatively small decrease of the NV 0 fluorescence by assuming that simultaneously to the NV 0 to NV − conversion, new NV 0 centres are created from non-fluorescent positively charged NV + centres. As previously reported for H-terminated diamond surfaces in contact with air [14] , the relative population of charge states of the NV centres depends on the implantation dose and is shifted to more negative charge states for increasing dose. This is illustrated in Fig. 2b–d , which present difference spectra at varying implantation doses. In regions of high implantation dose ( ∼ 10 13 cm −2 , Fig. 2b ), most NVs are in the negatively charged NV − state, with few NVs being neutrally charged. A change of the gate voltage shifts this distribution and induces an increase of NV − fluorescence at the expense of the NV 0 component. In regions of low implantation dose (approximately 10 11 cm −2 , Fig. 2d ), the NV − state is not populated at all and only few centres are in the neutral state NV 0 , whereas most centres discharge into a non-fluorescent state, potentially NV + . Changing the gate voltage shifts this equilibrium between NV 0 and NV + . In the spectra, this manifests itself as a rise of the NV 0 component, probably at the expense of an invisible NV + component. For medium implantation dose (approximately 10 12 cm −2 , Fig. 2c ), the spectrum is an interpolation between Fig. 2b, d . We observe a rise of the NV − component, which is not accompanied by a decrease in the NV 0 component. We tentatively attribute this latter observation to the NV 0 population being simultaneously replenished from an invisible NV + population. Switching behaviour of individual NV centres We were able to demonstrate electrical control of the charge state not only of an ensemble of NV centres, but even on a single-centre level in a sparsely implanted region ( Fig. 3a , nitrogen implantation dose ∼ 10 10 cm −2 , similar to region (1) in Fig. 1c ). As shown in Fig. 2e , centres exhibit the characteristic spectrum of NV 0 . 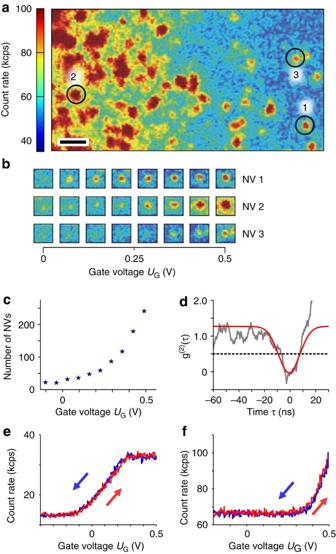Figure 3: Charge state control of single NV centres. (a) Fluorescence image of a 5 keV spot in a hydrogenated region at gate potentialUG=0.5 V, bar indicates 1 μm. (b) Selected centres at various gate voltages. (c) Number of NV centres visible in the scanned region of (a) at different gate voltages. (d) Photon statistics g(2)(τ) measured on a single centre (background corrected,UG=0.5 V). (e,f) Gate-voltage dependence of the fluorescence intensity of two single NV centres. Figure 3: Charge state control of single NV centres. ( a ) Fluorescence image of a 5 keV spot in a hydrogenated region at gate potential U G =0.5 V, bar indicates 1 μm. ( b ) Selected centres at various gate voltages. ( c ) Number of NV centres visible in the scanned region of ( a ) at different gate voltages. ( d ) Photon statistics g (2) (τ) measured on a single centre (background corrected, U G =0.5 V). ( e , f ) Gate-voltage dependence of the fluorescence intensity of two single NV centres. Full size image Upon increasing the gate voltage towards more positive values, an increasing number of NV centres become visible ( Fig. 3b, c ), most of which are single centres as confirmed by measuring photon statistics g (2) (τ) ( Fig. 3d ). To study the switching process of a single centre in more detail, we monitored the fluorescence intensity of several single centres as a function of the applied gate voltage ( Fig. 3e, f ). Fluorescence sets in above a certain threshold voltage and grows for increasingly positive voltages, as the centre is transferred from a non-fluorescent state, possibly NV + , into the fluorescent state NV 0 . We observed that the exact value of the threshold voltage differs among the centres ( Fig. 3e, f ). As we have discussed elsewhere [14] , the charge state of NV centres can be described in terms of the position of the charge transition level with respect to the Fermi level ( E F ). In our experiments, the applied gate voltage controls E F at the diamond surface ( Fig. 1b ). As a result, a band bending is imposed, so that the energy difference between charge transition level and Fermi level for a given centre depends on its distance to the surface. We numerically modelled this effect and calculated the band structure of diamond in contact with an electrolyte and, based on it, the charge state of the NV centres as described previously [14] (see Methods section). A voltage U G can be applied between the diamond substrate and an external reference electrode in the electrolyte. 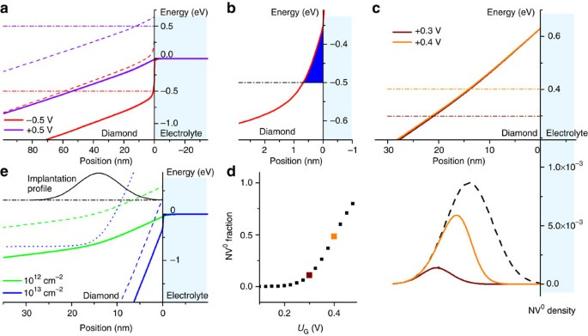Figure 4: Simulation of the energy band structure of H-terminated diamond in contact with an electrolyte. (a) AtUG=−0.5 V (red), the Fermi levelEF(dash-dotted line) crosses the charge transition level NV+/0(dashed line) much deeper in the diamond as compared withUG=+0.5 V (blue). (b) At negativeUG, the Fermi level lies below the VBM (solid line) in the surface region, inducing a two-dimensional hole gas (2-DHG; blue area). (c) Energy band schematic showing the intersection of the Fermi level with the NV+/0level atUG=0.3 V andUG=0.4 V. The density profile of neutrally charged NV is shown in comparison with the implantation. (d) Simulated fraction of neutrally charged NV versus the gate voltage. (e) VBM and the NV+/0(dashed lines), as well as the NV0/−charge transition levels (dotted line), are shown for two different implantation dose (1012and 1013cm−2). The background nitrogen concentration is 50 p.p.b. The implantation density profile for 10 keV is shown for reference. Figure 4a illustrates the resulting energy band structure of H-terminated diamond in contact with an electrolyte for two different voltages: U G =±0.5 V. The charge transition level of NV +/0 is set to 0.65 eV above the VBM to best fit the experimental results. This is in the region of the respective energy level reported in literature [23] , [27] . The energies are plotted such that the potential in the electrolyte is zero. For U G =−0.5 V, the simulations reproduce the two-dimensional hole gas at the diamond surface (blue area in Fig. 4b ), where the Fermi level has been pushed below the VBM. As the charge transition level follows the VBM with a constant energy distance, it will intersect with the Fermi level only deeper in the diamond. This marks the position where an NV centre will change its charge state upon a small variation of the applied voltage U G (see Fig. 1b ). The closer the NV centre to the surface, the more positive gate voltage is required to change its charge state from NV + to NV 0 . The varying threshold voltages observed for different NV centres ( Fig. 3e, f ) can therefore be interpreted as a result of the different distances of the NV centres to the surface or different local environments. An NV centre implanted deep in the diamond crystal would show a charging from NV + to NV 0 (onset of fluorescence) at more negative gate voltages, compared with a shallow centre. Figure 4c shows a detail of the energy band structure for two different gate voltages, 0.3 and 0.4 V, illustrating the intersection between E F and the charge transition NV +/0 . In addition, the implantation profile is compared with the density profile of NV 0 at these two gate voltages, indicating that the NV 0 charge state can only exist in those regions where the Fermi level is above the charge transition level NV +/0 . Integrating the density profile of NV 0 for different applied potentials and comparing it to the total number of implanted NV ( Fig. 4d ), the calculated NV 0 fraction nicely reproduces the experimental gate dependence shown in Fig. 3c . Figure 4: Simulation of the energy band structure of H-terminated diamond in contact with an electrolyte. ( a ) At U G =−0.5 V (red), the Fermi level E F (dash-dotted line) crosses the charge transition level NV +/0 (dashed line) much deeper in the diamond as compared with U G =+0.5 V (blue). ( b ) At negative U G , the Fermi level lies below the VBM (solid line) in the surface region, inducing a two-dimensional hole gas (2-DHG; blue area). ( c ) Energy band schematic showing the intersection of the Fermi level with the NV +/0 level at U G =0.3 V and U G =0.4 V. The density profile of neutrally charged NV is shown in comparison with the implantation. ( d ) Simulated fraction of neutrally charged NV versus the gate voltage. ( e ) VBM and the NV +/0 (dashed lines), as well as the NV 0/− charge transition levels (dotted line), are shown for two different implantation dose (10 12 and 10 13 cm −2 ). The background nitrogen concentration is 50 p.p.b. The implantation density profile for 10 keV is shown for reference. Full size image In principle, application of an even higher gate voltage should allow to raise the Fermi level even above the NV 0/− level, and hence charge these single centres into the NV − state. We were not able to demonstrate this experimentally, as the range of accessible gate voltage is limited by the risk of surface oxidation. However, the NV 0/− level could be reached in regions of higher implantation dose. The key idea can be understood from Fig. 4e . The strength of the band bending in the diamond depends on the density of impurities, which can be varied by the dose of implanted nitrogen. At a fixed depth, a stronger band bending lowers all energy levels with respect to the Fermi level and is therefore indistinguishable from an increase of the gate voltage. Thus, a lower gate voltage allows to shift the Fermi level across the NV 0/− level. Figure 4e illustrates this effect for two cases of low and high implantation dose. An implantation dose of 10 12 cm −2 induces a weaker band bending. Here, centres very close to the surface (see implantation profile in Fig. 4e ) remain in their positive charge state. The rest of the implanted centres will be neutrally charged as E F is above the NV +/0 level. For a higher implantation dose of 10 13 cm −2 , the band bending within the first 20 nm is strongly enhanced because of the additional nitrogen donors implanted close to the surface. Therefore, no NV centres will be positively charged and some (up to a depth of around 10 nm) will be in the neutral state. At this depth, the Fermi level rises even above the NV 0/− charge transition level, so that all deeper centres will be negatively charged. It is by means of this effect that we were able to demonstrate switching between NV 0 and NV − in Fig. 2b . By performing the experiment at high implantation dose ( ∼ 10 13 cm −2 ), we place ourselves in the 'blue' scenario of Fig. 4e . The strong band bending associated to this high implantation dose implies that most NV centres remain negatively or neutrally charged. Here, a change of U G from −0.5 to 0.5 V increases the NV − fluorescence at the expense of the NV 0 component as seen in Fig. 2b . As the dose is lowered ( Fig. 2d, e ), we place ourselves in the 'green' scenario of Fig. 4e where the band bending is weak. Under these conditions, only the NV +/0 level intersects with E F within the implantation region, and a shift of the gate voltage mainly causes the conversion between NV 0 and NV + . As the NV −/0 level is situated higher above the valence band, the crossing between E F and this charge transition level is expected further away from the diamond surface where no NV centres are implanted. Thus, a much larger gate voltage would be necessary to shift this crossing close to the implantation region in the vicinity of the surface. Because of the risk of surface oxidation, this is experimentally not accessible, so that single negatively charged NV centres cannot be observed in our present setting. In conclusion, we have shown that an electrical manipulation of the charge state of shallow implanted NV centres below hydrogenated diamond surfaces is possible by using an external gate electrode. Ensembles of NV centres can be switched reversibly between NV 0 and NV − by the gate voltage, whereas the charge state of single NV centres can be switched between positive and neutral. Numerical simulations, modelling the effect of the gate electrode on the diamond band structure, provide a quantitative description of the experimental results. These findings offer a first way to reversibly control the charge state of the NV centres in an extremely versatile manner, providing an important tool for the use of single NV centres for diamond-based spintronics or sensing applications. Furthermore, our results open the way to study formerly unstable or unknown charge states like NV 0 and the positively charged NV + , for which several applications have already been proposed [22] . Sample preparation Experiments were conducted on electronic grade, synthetic, single-crystalline diamonds with a nitrogen concentration specified below 5 p.p.b. (purchased from Element Six Ltd). Two samples were used with NV centres created by the implantation of 15 N + ions with an energy of 5 and 10 keV per ion, respectively, at an implantation angle of 0°, followed by thermal annealing at 800 °C [29] . The average implantation depths can be estimated by SRIM calculations [26] to be 7 and 14 nm. The ion beam was defocused to vary the implantation dose over three orders of magnitude (10 10 –10 13 ions per cm 2 ). This allows experiments on either single optically resolved NV centres or on densely implanted regions (regions 1 and 2 in Fig. 1c ). Samples were patterned with oxygen (O)- and hydrogen (H)-terminated regions (see Fig. 1c ) by photolithography and plasma treatment in a microwave-assisted plasma reactor. The O-terminated regions serve as reference areas to determine the local implantation density. The H-terminated surface was electrically contacted and isolated with a chemically stable silicone rubber. A potassium phosphate buffer (10 mM K-PBS buffer, 50 mM KCl, pH7) was used as a gate electrolyte and immersion liquid, and showed no fluorescence upon laser excitation. The electrolyte was contacted with a Pt electrode, and gate voltages from 0.5 to −0.5 V were applied between the diamond surface and the electrode. No voltages outside this potential window were applied to avoid electrochemical oxidation of the surface. Experimental setup Optical measurements were performed with a home-built confocal microscope. A continuous-wave, diode-pumped, frequency-doubled Nd:YAG laser at a wavelength of λ =532 nm was used to excite the NV centres. The fluorescence signal was filtered by a 650-nm longpass filter and recorded by an avalanche photodiode or, alternatively, filtered by a 560-nm longpass filter and routed to a spectrometer (Acton 2300, Princeton Instruments with Pixis 100B camera). Modelling and numerical simulations The model for numerical simulations of the experimental results is based on the assumption that the NV centre exists in one of three charge states: negative (NV − ), neutral (NV 0 ) and positive (NV + ). We assume that photoexcitation of these centres into highly excited states near the conduction band leads to rapid thermalization. The charge state is then determined exclusively by the relative position of the Fermi level with respect to the charge transition levels. The fluorescence intensity of NV − and NV 0 is a measure of the ground state occupation of these charge states. In this way, we reduce the complex multi-level system of all ground, excited and metastable states of all defects in the diamond to an effective three-level system of NV charge transition states [23] , whose equilibrium occupation is governed exclusively by the position of the Fermi level. By assuming thermal equilibrium, we neglect that photoexcitation could lead to a non-equilibrium distribution. In particular, traps above the Fermi level could be populated upon laser excitation. However, these traps are likely to thermalize with their local environment on a fast timescale. We consider this effect to be small and therefore use the thermal equilibrium model in which the population of states is exclusively governed by the position of the Fermi level. Although the assumption of thermal equilibrium is a nontrivial approximation, we have so far not seen a departure from this model, neither in the results of this work nor in previous results [14] . Numerical simulations were performed using the nextnano software [3] . Nextnano is a semiconductor device simulation tool developed at the Walter Schottky Institute to predict and understand a wide range of electronic and optical properties of semiconductor structures and nanostructures [30] . It can calculate the electronic band structure, the carrier density and the electrostatic potential of a one-, two- or three-dimensional device consisting of different materials in a self-consistent manner. A detailed description of the nextnano simulation techniques has been published [29] . The single band effective mass Schrödinger equation is coupled to the Poisson equation via the charge density as described by the wave functions in the diamond, which then is solved numerically in a self-consistent manner. The occupation of the subbands and defect levels in the band gap is determined by the energetic position relative to the Fermi level. The diamond is modelled in contact with an electrolyte and a gate voltage U G is applied between the diamond and an external reference electrode in the electrolyte. We use the Dirichlet boundary condition for the electrostatic potential in the bulk electrolyte and the Neumann boundary condition (vanishing electric field) deep in the diamond. The parameters used in the nextnano simulation are listed in Table 1 . Table 1 Parameters used in the nextnano simulation. Full size table How to cite this article: Grotz, B. et al . Charge-state manipulation of qubits in diamond. Nat. Commun. 3:729 doi: 10.1038/ncomms1729 (2012).